Amide nitrogen pyramidalization changes lactam amide spinning Although cis - trans lactam amide rotation is fundamentally important, it has been little studied, except for a report on peptide-based lactams. Here, we find a consistent relationship between the lactam amide cis/trans ratios and the rotation rates between the trans and cis lactam amides upon the lactam chain length of the stapling side-chain of two 7-azabicyclo[2.2.1]heptane bicyclic units, linked through a non-planar amide bond. That is, as the chain length increased, the rotational rate of trans to cis lactam amide was decreased, and consequently the trans ratio was increased. This chain length-dependency of the lactam amide isomerization and our simulation studies support the idea that the present lactam amides can spin through 360 degrees as in open-chain amides, due to the occurrence of nitrogen pyramidalization. The tilting direction of the pyramidal amide nitrogen atom of the bicyclic systems is synchronized with the direction of the semicircle-rotation of the amide. Rotation of amides is of fundamental importance [1] , [2] , being involved in a wide range of structural phenomena ranging from protein folding [3] , [4] , [5] , [6] to the conformational multiplicity of cyclic peptides [7] , [8] , [9] , [10] , [11] . In the case of cyclic amides (lactams), rotation of the amide is influenced by the intervening chain length and nature of the rotatable bonds. If a lactam amide bond could spin through 360 degrees as in open-chain amides, a simple correlation between the ratio of amide trans/cis isomers and the rotational rate(s) between trans and cis amide conformers should be observed, e.g., as the rotation rate from trans to cis isomers increases, the ratio of cis isomer increases. While there have been few studies of the rotation rate of lactam amides, the rotation rate of α−proline amide upon intramolecular disulfide bond formation between two flanking cysteine (Cys) residues was reported to show an inconsistent dependency of cis - trans isomer ratios and rates of cis - trans interconversion on chain length. This is probably because spinning of the amide bond is discontinuous and also because the energy barrier of amide rotation is relatively high (~20 kcal/mol) [12] , [13] , [14] . Therefore, this observation suggested that the rotation of lactam amide is restricted [15] , [16] , [17] , and as a general trend, the amide bond in lactams cannot spin through 360 degrees, probably due to ring coiling (Fig. 1a ). For example, a simple N-methyl tertiary amide lactam, a medium-ring-sized 1-methylazacycloundecan-2-one (11-membered ring) ( S-A , Supplementary Fig. 1 ) and a simple secondary amide lactam, a large-ring-sized 1-azacyclononadecan-2-one (19-membered ring) ( S-B , Supplementary Fig. 2 ), exhibited discontinuous spinning of the lactam amide bond, not through 360° (see also Supplementary Fig. 3 ). Fig. 1 Lactam amide rotations. a Hindered rotation of coiled lactam amides. b Nitrogen pyramidalization of tertiary amide lactams of 7-azabicyclo[2.2.1]heptane. c Equilibrium of trans and cis amides in the bicyclic N-pyramidal lactam. d Spinning of N-pyramidal lactam through 360 degrees Full size image On the other hand, while non-planar amides have been studied intensively [18] , [19] , [20] , [21] , [22] , [23] , [24] , [25] , [26] , their characteristic structural features and the consequent reduction of amide rotational barriers have been little utilized in molecular architecture, mainly because of the instability of the amide bond under conventional transformation conditions. However, examination of tertiary amides of 7-azabicyclo[2.2.1]heptane has shown that this bicyclic system induces nitrogen pyramidalization (Fig. 1b ) [27] , and these amides are stable enough to be subjected to further transformations [28] . The rotational barriers of amide cis-trans isomerization of nitrogen-pyramidal amides are reduced in solution (~17 kcal/mol), indicating more facile amide rotation as compared with conventional planar amides (>20 kcal/mol). Inversion of the amide nitrogen atom is a low-energy process (calculated activation energy: less than 3 kcal/mol), and nitrogen pyramidalization is also a facile process [27] , [29] . Further, derivatives bearing a carboxylic acid functionality at the C 2 -position can be regarded as conformation-constrained β-proline surrogates. In these bicyclic β-proline surrogate 7-azabicyclo[2.2.1]heptane-2-carboxylic acids (Fig. 1c ), it is shown that the presence of the bridgehead substituent at the C 4 -position completely biases the amide cis - trans equilibrium to one side ( trans amide), irrespective of solvent [30] , [31] , [32] . This led us to consider that side-chain stapling of the bicyclic amide dimer would affect the thermodynamics and kinetics of non-planar amide lactam rotation in a very definite manner (Fig. 1c ). Therefore, we expected that this bicyclic system would provide a suitable scaffold to examine the stapling length dependency of lactam amide ratio and rotation (see below). Here, we show a simple relationship; i.e., a consistent increase of trans ratio in accordance with a consistent deceleration of amide trans to cis rotation, together with concomitant acceleration of amide cis to trans rotation, as the side-chain staple length is increased in bicyclic dimers, eventually affording a very large dynamic range of variation in amide cis - trans ratios, extending to complete inversion of the amide cis - trans equilibrium, depending upon the side-chain staple length (Fig. 1d ). Analysis of amide cis-trans isomerization We used ring-closing metathesis (RCM) [33] , [34] to staple model bridgehead-substituted bicyclic dimers with various lengths of alkyl side chain (Fig. 2 ). Cyclic dimer lactams ( 16–20 ) with linkers of different lengths were synthesized as racemic mixtures (for details, see Supplementary Methods). The RCM reactions of 1–5 , which are Boc-protected open-chain model dimers with alkenyl side chains of various lengths, were performed using the Grubbs I catalyst to afford stapled olefin products 6–10 as mixtures of E -olefins and Z -olefins in good yields (Supplementary Fig. 18 ). Hydrogenation of the alkenes gave N-Boc saturated compounds 11–15 , respectively (Supplementary Fig. 18 ). Some of the structures were confirmed by means of X-ray crystallographic analyses (see below). Fig. 2 Lactams containing two 7-azabicyclo[2.2.1]heptane bicyclic units. Stapling of model bridgehead-substituted bicyclic dimers with various lengths of alkyl side chain by ring-closing metathesis (RCM) and hydrogenation Full size image The Boc group was removed by treatment of 11–15 with TFA, followed by base treatment to give the dimer free amines ( 16(C8) , 17(C9) , 18(C10) , 19(C11) , and 20(C12) ) (for chemical structures, see Fig. 2 ), where the number C n indicates the number ( n ) of carbons between two ether oxygen atoms of the linker. The amide cis/trans ratio of the dimer lactams ( 16(C8) - 20(C12) ) was estimated from the NMR spectra in CD 2 Cl 2 . 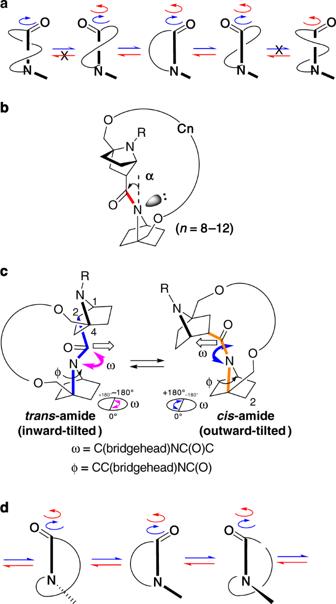Fig. 1 Lactam amide rotations.aHindered rotation of coiled lactam amides.bNitrogen pyramidalization of tertiary amide lactams of 7-azabicyclo[2.2.1]heptane.cEquilibrium oftransandcisamides in the bicyclic N-pyramidal lactam.dSpinning of N-pyramidal lactam through 360 degrees We found that the ratio changed dramatically depending upon the linker length (Table 1 ). The open-chain amide analogue 1–5 (which can be regarded as equivalent to a cyclic molecule with an infinite linker length) takes exclusively the trans -amide structure (Table 1 ). The ratio of cis -amide in the lactam analogs is increased as the linker length is decreased and the ratio changes from predominantly trans ( 20(C12) , 94% trans , K c/t = 0.06) to almost exclusively cis ( 16 (Z) -NH(C8)(Z-olefin) , 99.9% cis , K c/t > 999) (Table 1 ). X-Ray crystallographic analysis of the synthetic intermediate unsaturated derivatives provided supporting evidence for the structural assignments (see below, Supplementary Figs. 14 – 16 ). As the chain length decreased, the energy difference between cis and trans lactam amides changed ( ΔΔG cis-trans = ΔG cis –ΔG trans , see Table 1 ): ΔΔG cis-trans (in CD 2 Cl 2 ); 19(C11) : + 1.08 kcal/mol ( trans more stable than cis ); 18(C10) : + 0.59 kcal/mol ( trans more stable than cis ); 17(C9) : −1.08 kcal/mol ( cis more stable than trans ) (Table 1 ): cis structure became more stable than trans structure. Also, there is a clear difference in the preference for trans - or cis -amide between lactams 17(C9) and 18(C10) . We found that 17(C9) and 18(C10) exhibit similar trans/cis ratios in CD 2 Cl 2 ( 17 : 14/86; 18 : 73/27) and protic CD 3 OD ( 17 : 24/76; 18 : 77/23), showing small dependency of solvent polarity on cis/trans isomer distribution. Table 1 Equilibrium constants of amide cis-trans isomerization at −50 °C Full size table Chain-length-dependent amide rotation kinetics The rotational kinetics of the amide bond of the bicyclic dimer with different linker lengths ( 16(C8) , 17(C9) , 18(C10) and 19(C11) ) was estimated by means of exchange spectroscopy (EXSY) [35] , [36] , [37] , [38] , [39] (Fig. 3a, b ). We measured the kinetics of 17(C9) , 18(C10) , and 19(C11) in CD 2 Cl 2 , and 16(C8) , 17(C9) , and 18(C10) in CD 3 OD (Fig. 3c, d ). The EXSY spectra were recorded with six mixing times ( T m ) of 20, 40, 60, 100, 200, and 300 ms at 215.4 K, 217.9 K, 220.4 K, 222.9 K, and 225.4 K in CD 2 Cl 2 and with six mixing times ( T mix ) at 222.8 K, 226.8 K, 230.6 K, 234.4 K, and 238.2 K in CD 3 OD. The signal intensities of the four peaks due to one pair of exchanging bridgehead protons were obtained from the peak heights (Fig. 3a ): I tt is the peak intensity of the auto peak of H 1 in the trans conformation (i.e., H 1 t ), I cc is that of the auto peak of H 1 in the cis conformation (i.e., H 1 c ), I tc is that of the cross peak from trans to cis conformation, and I ct is that of the cross peak from cis to trans conformation. (Fig. 2 ). The assignments were confirmed by the observation of NOE between H 1 c and H 2 c (Supplementary Figs. 4 – 7 ). The exchange rate ( k t → c ) from trans to cis conformation and that ( k c → t ) from cis to trans conformation at each temperature were estimated by fitting to a modified version of the theoretical equation reported previously (Fig. 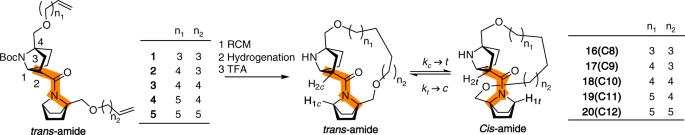Fig. 2 Lactams containing two 7-azabicyclo[2.2.1]heptane bicyclic units. Stapling of model bridgehead-substituted bicyclic dimers with various lengths of alkyl side chain by ring-closing metathesis (RCM) and hydrogenation 3b, Table 2 , Supplementary Figs. 8 – 13 ) [39] , [40] . The free energies of rotation (∆ G t → c ‡ and ∆ G c → t ‡ ) were obtained from the enthalpy of activation (∆ H ‡ ) and the entropy of activation (∆ S ‡ ), which were derived from the slope and intercept of the Eyring plot of the rate against temperature (Table 2 ). Fig. 3 Kinetic studies of lactam amide rotations. a EXSY spectrum of 18(C10) in CD 2 Cl 2 at −50.3 °C with a mixing time of 50 ms. b Plots of the signal intensities of 18(C10) versus the mixing time (−50.3 °C). Solid lines indicate the best fit of the data to the theoretical equation. c Dependency of isomerization rate of trans to cis amide isomers on the staple length. d Dependency of isomerization rate of cis to trans amide isomers on the number of chain carbon atoms. Blue square and blue line: the rotation rate in CD 2 Cl 2 at −50.3 °C; red triangle and red line: the rotation rate in CD 3 OD at −42.6 °C. Blue bar: the rotation barrier (Δ G ‡ (−50.0 °C) ) in CD 2 Cl 2 , red bar: Δ G ‡ (−50.0 °C) in CD 3 OD Full size image Table 2 Rate constants and activation parameters for amide cis-trans isomerization Full size table The rotation rates in CD 3 OD were apparently smaller than those in CD 2 Cl 2 , suggesting a possible contribution of solvation effects in the rotation process, such as entropy, polarity and viscosity of the solvent (Table 2 ). The rotation rate k t → c showed a consistent decrease along the sequence from 16(C8) to 18(C10) (in CD 3 OD) and from 17(C9) to 19(C11) (in CD 2 Cl 2 ) (Fig. 3c ). On the other hand, the rotation rate from cis to trans isomer ( k c → t ) showed a small but consistent increase along the sequence from 16(C8) to 18(C10) (in CD 3 OD) and from 17(C9) to 19(C11) (in CD 2 Cl 2 ) (Fig. 3d ). Finally, as the number of ring carbon atoms ( C n ) increases along the sequence from 16(C8) to 19(C11) , the magnitude of the rotation rate from cis to trans isomer ( k c → t ) overwhelms that of the rotation rate from trans to cis isomer ( k t → c ), which is consistent with the large dynamic range of variation in amide cis - trans ratios, extending to complete inversion of the cis - trans equilibrium from cis isomer to trans isomer. In fact, these changes in the rotation rate ( k ) are consistent with the changes in the free energy of rotation (∆ G t → c ‡ and ∆ G c → t ‡ ): ∆ G t → c ‡ ( trans to cis ) decreased with reduction in the size of the stapling ring (Fig. 3c and Table 2 ), while ∆ G c → t ‡ ( cis to trans ) showed a slight increase (Fig. 3d and Table 2 ). The obtained rotational barriers of trans to cis isomer (Δ G t → c ‡ ) (at 223.2 K) for 17(C9) - 19(C11) ranged from 11.4 kcal/mol, 12.3 kcal/mol to 12.9 kcal/mol in CD 2 Cl 2 , and those for 16(C8) - 18(C10) ranged from 12.1 kcal/mol, 12.3 kcal/mol to 13.0 kcal/mol in CD 3 OD (Table 2 ). These values are significantly reduced compared to those of the parent open-chain bicyclic amide ( Ac-Ah2c-NHMe ) (ca. 17 kcal/mol) [40] . As the linker becomes shorter, the enthalpy of activation (Δ H ‡ ) decreases and entropic ordering is increased. We also saw a similar trend in CD 3 OD. Different ring size effects on cis and trans amide structures In order to examine the ring size of the experimentally studied systems, we calculated the energy-minimum structures of lactams 16 – 19 by means of DFT methods (see Supplementary Data and Supplementary Methods ). The DFT calculated structures of trans -amide structures showed that, as expected, decrease in the stapling chain number ( n ) is accompanied with decrease of the ring size, as exemplified by a large decrease of the distance between the two ether oxygen atoms ( d o-o ), which is related to the radius of the ring ( trans forms: 16(C8) : 7.01 Å; 17(C9) : 7.76 Å; 18(C10) : 7.94 Å; 19(C11) : 8.24 Å) (Fig. 4a ). On the other hand cis -amide structures showed a small change in the ring size as exemplified by the distance ( d o-o ) between the two ether oxygen atoms in the ring, and there was a fluctuation at 18(C10) : the cis forms: 16(C8) : 6.01 Å; 17(C9) : 6.21 Å; 18(C10) : 6.15 Å; 19(C11) : 6.34 Å) (Fig. 4b ). From the observed cis/trans ratio (Table 1 ), a short ring linking two adjacent bridgehead groups stabilizes cis amide structures, while the cis amide was destabilized by increase of chain length. Fig. 4 DFT-optimized structures of 16(C8) - 19(C11) . a DFT-optimized trans -isomers of 16(C8) - 19(C11) . b DFT-optimized cis -isomers of 16(C8) - 19(C11) . The distance between the ether oxygen atoms in the linker is shown in blue. Brown/gray: carbon atom; blue: nitrogen atom; red: oxygen atom. All hydrogen atoms are omitted for clarity Full size image The dependency of the rotation rate from trans to cis isomer ( k t → c ) on the chain length can be accounted for by the fact that the increase of the ring size (e.g., elongation of d O-O ) led to increase of the trans ratio (Table 1 ), which indicates that increase of the ring size stabilized the trans amide structure, probably due to release of the trans -lactam ring strain (Fig. 4a ). When the initial trans structure was stabilized, the activation energies for amide rotation to reach the TS structure may be increased, and therefore amide rotation becomes less feasible, i.e., the rotation rate from trans to cis isomer ( k t → c ) becomes smaller. For 18(C10) the change in the rotation rate fluctuated slightly (Fig. 3d , in CDCl 3 ), probably because there is a structural inconsistency in cis 18(C10) due to shrinkage of the ring size at 18(C10) ( d O-O : 6.15 Å) as compared with 17(C9) ( d O-O : 6.21 Å), in spite of the increased size of the carbon chain (Fig. 4b ). Therefore, although there is a fluctuation, there is a tendency that the rotation rate from cis to trans isomer ( k c → t ) increases (Fig. 3d ) as the stable cis isomer become more unstable along the sequence from 16(C8) to 19(C11) , judging from the observed decrease in the cis ratio (Table 1 ). This destabilization of the cis amide structure upon increase in the ring size is probably due to the increase in strain to maintain the fixed distance between the two ether oxygen atoms. The extension of these two ether linkages is forced to take a parallel direction, as seen in the crystal structures of the cis amides, i.e., cis -C7-N-Boc and cis −6Z-C8-N-Boc (Fig. 5a, b ). Fig. 5 ORTEP drawings (50% probability) of the crystal structures of some derivatives. a The crystal structure of N -Boc derivative of C7 in the cis amide form. b The crystal structure of N -Boc derivative of 6 ( Z ) ( C8 ) in the cis -amide form, and c the crystal structure of N -tosylated derivative of 8 ( E ) ( Ts-8 ( E )( C10 )) in the trans -amide form. All three structures were crystallized as racemates in centrosymmetric space groups. DFT-optimized structures are also shown. The distance between the ether oxygen atoms in the linker is shown in blue. Brown/gray: carbon atom; blue: nitrogen atom; red: oxygen atom. All hydrogen atoms are omitted for clarity Full size image Tilting direction of the pyramidal nitrogen atom While the crystal structures (Fig. 5a, b, c ) are different from the real system ( 16 – 19 ) due to the presence of the unsaturation of the alkyl chain and N-substitution (Boc or Ts), it seemed that the amides of the ground states ( trans and cis isomers) were tilted in the opposite direction to the bridgehead substituent; this is particularly apparent in the cases of the C8 ( cis −6(Z)(C8)-N-Boc ) and C10 ( trans −8(E)(C10)-N-Ts ) analogues (Fig. 5b, c ). The DFT-optimized structures, starting from the X-ray structures of cis -C7-N-Boc , cis −6(Z)-C8-N-Boc , and trans −8(E)(C10)-N-Ts , supported this trend (Fig. 5 a–c). The tilting of the amide on the same side of the bridgehead substituent induced significant destabilization (calculated as more than 60 kcal/mol). The calculated averaged tilt angles ( α ) were 25.0° and 20.7° for the trans -ground state and cis -ground state, respectively (Fig. 1b and Fig. 4a, b ). These structural features are a consequence of the facile nitrogen pyramidalization of the bicyclic lactam amide. Computational evaluation of the lactam amide rotation DFT calculation was performed to identify features of the rotational process. As a result of an extensive search of amide rotation processes, transition structures for amide rotation of the 2( S )-enantiomers of 17(C9) , 18(C10) , and 19(C11) were identified (Supplementary Fig. 53 , Supplementary Methods and Supplementary Data ); these may represent one of the lowest-energy processes. Both the magnitude of the rotational barrier and the relative stability of cis-trans rotamers coincided well with the experimental values. The calculated values of free energy of rotation from trans to cis (∆ G ‡ t → c ) in CH 2 Cl 2 at 25 °C were 9.6 kcal/mol, 12.7 kcal/mol and 13.6 kcal/mol in 17(C9) , 18(C10) , and 19(C11) , respectively (Supplementary Table 1 ). On the other hand, the calculated values of free energy of rotation from cis to trans (∆ G ‡ c → t ) in methanol at 25 °C were 14.5 kcal/mol, 11.9 kcal/mol and 11.8 kcal/mol in 16(C8) , 17(C9) , and 18(C10) , respectively (Supplementary Table 2 ). Therefore, the computations reproduced the tendency that the rotational barrier, especially ∆ G ‡ c → t (Supplementary Table 2 and Fig. 3d ), decreases as the alkyl linker is elongated. Metadynamics simulations [41] of bicyclic amides 17(C9) and 19(C11) (Fig. 6a and Supplementary Fig. 54 ) revealed that the present system is an example in which 360 degree rotation of lactam nitrogen can occur owing to nitrogen pyramidalization: in principle, lactam amide rotation (dihedral angle ω , ∠ C(bridgehead)NC(O)C in Fig. 1c ) is restricted to a south semicircle-rotation angle (e.g., ω:0° to +180°) or a north semicircle-rotation angle (e.g., ω :−180° to 0°) ( Fig. 1c ) with respect to the amide dihedral angle (ω) due to the ring coiling (see Fig. 1b ), but in the present case ( 17(C9) and 19(C11) ), lactam amide rotation can undergo continuous north semicircle-rotation with inward-tilted amide nitrogen pyramidalization (dihedral angle ϕ = 150° in Fig. 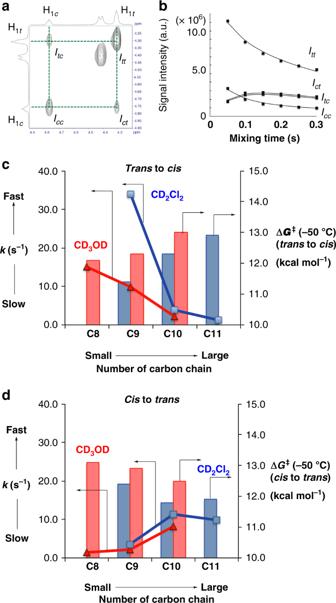Fig. 3 Kinetic studies of lactam amide rotations.aEXSY spectrum of18(C10)in CD2Cl2at −50.3 °C with a mixing time of 50 ms.bPlots of the signal intensities of18(C10)versus the mixing time (−50.3 °C). Solid lines indicate the best fit of the data to the theoretical equation.cDependency of isomerization rate oftranstocisamide isomers on the staple length.dDependency of isomerization rate ofcistotransamide isomers on the number of chain carbon atoms. Blue square and blue line: the rotation rate in CD2Cl2at −50.3 °C; red triangle and red line: the rotation rate in CD3OD at −42.6 °C. Blue bar: the rotation barrier (ΔG‡(−50.0 °C)) in CD2Cl2, red bar: ΔG‡(−50.0 °C)in CD3OD 6a and Supplementary Fig. 54, B to A )) and at the same time continuous south semicircle-rotation with outward-tilted amide nitrogen pyramidalization (dihedral angle ϕ = 100° in Fig. 6a and Supplementary Fig. 54, A to B’ ). Similar diagrams were obtained in the cases of 16(C8) and 18(C10) (for example, Supplementary Fig. 55 ). X-Ray crystallographic analysis shows that 6 ( Z )( C8 ) takes cis -amide structure with outward-tilted amide nitrogen pyramidalization, consistent with the simulated cis amide structures d in 17(C9) (Fig. 6a ) and 19(C11) (Supplementary Fig. 54 ), respectively. In contrast, the trans amide of the N -tosylated derivative of 8 ( E) ( Ts-8 ( E )( C10 )) (crystal structure, Fig. 5c ) takes the structure with inward-tilted amide nitrogen pyramidalization, which is consistent with the simulated trans amide structures a in 17(C9) (Fig. 6a ) and 19(C11) (Supplementary Fig. 54 ), respectively. The rotation is dual-directional. The difference between the energy barrier (~4 kcal/mol at b ) in north semicircle-rotation ( a → d , Fig. 6a : trans → cis ) and the energy barrier (~7 kcal/mol at e ) in south semicircle-rotation ( d → e , Fig. 6a : cis → trans ) is consistent with the difference in observed rotation speed ( k t → c > k c → t ) of 17(C9) (Table 2 ) . As already discussed, the DFT-calculated cis amides of 16(C8) - 19(C11) also show outward-tilted amide nitrogen pyramidalization (Fig. 4b ), while the DFT calculated trans amides of 16(C8) - 19(C11) show inward-tilted amide nitrogen pyramidalization (Fig. 4a ). Fig. 6 The landscape of lactam amide rotation. a Metadymamic simulations of bicycle lactam 17(C9) in chloroform at 300 K. Dashed lines indicate the rotational pathways. The tilting direction of the pyramidal nitrogen atom of the bicyclic systems is synchronized with the direction of the semicircle-rotation of the amide. b Metadymamic simulations of monocycle lactam 21( S -C9) in chloroform at 300 K. Dashed lines indicate the rotational pathways. Rotation of the lactam amide bond is restricted to a south semicircle-rotation angle (e.g., 0° to + 180°) Full size image On the other hand, metadynamics simulations of virtual monocyclic pyrrolidine amides ( 21( S -C9) and 22( S -C11) , Fig. 6b and Supplementary Fig. 56 ), in which the lower 7-azabicyclo[2.2.1]heptane is replaced with a monocyclic pyrrolidine derivative, show that one dihedral angle around the amide nitrogen atom is allowed, and the rotation with respect to the amide bond is restricted to a south semicircle-rotation angle (e.g., 0° to + 180°, Fig. 6b and Supplementary Fig. 56, A to B ): a north semicircle-rotation (e.g., angle ω : −180° to 0°, Fig. 6b and Supplementary Fig. 56, B’ to A ) is inhibited by the high activation barrier. The R -configuration model compounds (( 23( R -C9) and 24( R -C11) , Supplementary Figs. 57 and 58 ) showed similarly restricted amide rotation. Monocyclic pyrrolidine amides take a planar amide structure, so nitrogen pyramidalization is probably crucial for the 360-degree spinning of lactam amide. A similar restriction in the rotation was also found in the case of the replacement of the lower bicyclic amide with the simple non-cyclic N-methyl amide ( 25 (C-9) and 25 (C-11) , Supplementary Fig. 3 ), probably due to the planar amide. Our findings indicate that side-chain stapling of these bicyclic dimer amides results in monotonous relationships between the rotational rate between cis and trans lactam amide and the ratio of the cis / trans isomers, depending on the ring size: as the ring size of the stapled structure is increased, the rotational rate of trans to cis conformer is decreased and that of cis to trans conformer is increased, resulting in an increase in the trans/cis ratio. Complete inversion of the amide equilibrium, affording an extreme range of cis/trans ratios (approximately 1/0~0/1), depending on the linker length, was observed. Our observations and simulations are consistent with the idea that the present lactam amide can spin through 360 degrees due to the occurrence of nitrogen pyramidalization. The tilting direction of the pyramidal nitrogen atom of the bicyclic systems is synchronized with the direction of the semicircle-rotation of the amide (Fig. 1c and d). The present results provided a new insight into the amide rotation of lactams, which are a ubiquitous and divergent class of compounds. The rotational features of lactam amides observed here might be generalized and find applications in molecular design. Synthesis Details of synthesis are given in the Supplementary Methods and Supplementary Figs. 18 – 52 . Synthesis of 16(C8) To a solution of 11 (99.6 mg, 0.2030 mmol) in CH 2 Cl 2 (6 mL) was added TFA (1 mL), and the whole was stirred for 2 h at 0 °C. The reaction mixture was poured into 10% aqueous solution of Na 2 CO 3 . The whole was extracted with CH 2 Cl 2 , dried over Na 2 SO 4 , and evaporated. Column chromatography (CHCl 3 /MeOH = 15/1) gave compound 16(C8) (45.2 mg, 57%) as a white solid.　M.p. : 101.5 °C–102.0 °C. 1 H-NMR (CDCl 3 ): 4.699 (1 H, t, J = 5.2 Hz), 3.983 (1 H, d, J = 11.6 Hz), 3.658 (1 H, d, J = 11.2 Hz), 3.581–3.446 (6 H, m), 3.356 (1 H, dt, J = 4.8 Hz, 8.8 Hz), 3.311–3.254 (1 H, m), 2.20–1.20 (27 H, m). 13 C-NMR (CD 2 Cl 2 ): 170.73, 73.16, 72.04, 71.77, 70.14, 69.10, 67.97, 61.29, 56.79, 48.70, 35.79, 33.47, 32.43, 30.01, 29.06, 28.83, 28.76, 28.46, 28.21, 26.68, 26.21, 25.76. HRMS (ESI, [M + H]+): Calcd. For C 23 H 39 N 2 O 3 + : 391.2955, Found: 391.2963. Synthesis of 17(C9) To a solution of 12 (20.6 mg, 0.04082 mmol) in CH 2 Cl 2 (0.9 mL) was added 0.15 mL of TFA, and the whole was stirred for 1 h at 0 °C and 1 h at rt. 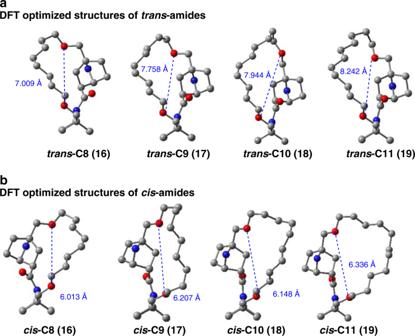Fig. 4 DFT-optimized structures of16(C8)-19(C11).aDFT-optimizedtrans-isomers of16(C8)-19(C11).bDFT-optimizedcis-isomers of16(C8)-19(C11). The distance between the ether oxygen atoms in the linker is shown in blue. Brown/gray: carbon atom; blue: nitrogen atom; red: oxygen atom. All hydrogen atoms are omitted for clarity The solvent was evaporated and 10% aqueous solution of Na 2 CO 3 was added to the residue to adjust the pH to 10. The aqueous layer was extracted with CH 2 Cl 2 , dried over Na 2 SO 4 , and evaporated. Column chromatography (CHCl 3 /MeOH = 30/1 to 20/1 to 10/1) and preparative TLC (CHCl 3 /MeOH = 20/1 and 0.1% Et 3 N) gave compound 17(C9) (8.6 mg, 52%) as a white solid. 1 H-NMR (CDCl 3 ): 4.682 (1 H, brs), 3.960 (1 H, d, J = 11.2 Hz), 3.813–3.792 (1 H, m), 3.88–3.72 (1 H, brs), 3.680 (1 H, d, J = 10.0 Hz), 3.610 (1 H, d, J = 10.0 Hz), 3.569–3.430 (4 H, m), 3.52–3.39 (1 H, m), 2.20–1.18 (28 H, m). 13 C-NMR (CDCl 3 ): 169.50, 72.54, 72.23, 71.81, 69.86, 69.69, 68.11, 61.15, 57.20, 46.61, 35.21, 33.05, 31.53, 30.12, 29.83, 29.27, 28.76, 28.56, 28.42, 27.60, 26.32, 25.27. HRMS (ESI, [M + H] + ): Calcd. For C 24 H 41 N 2 O 3 + : 405.3112, Found: 405.3125. Synthesis of 18(C10) To a solution of 13 (68.2 mg, 0.131 mmol) in CH 2 Cl 2 (3 mL) was added TFA (0.5 mL) and the whole was stirred for 4 h at 0 °C and 1 h at 10 °C. The reaction mixture was poured into 10% aqueous solution of Na 2 CO 3 . The whole was extracted with CH 2 Cl 2 , dried over Na 2 SO 4 . Then the solvent was evaporated. Column chromatography (CHCl 3 :MeOH = 30:1 to 20:1 to 10:1) and preparative TLC (CHCl 3 /MeOH = 16/1 and 0.2 % NEt 3 ) gave 18(C10) (52.3 mg, 95%) as colorless oil. 1 H-NMR (50 °C, CD 2 Cl 2 ): 4.517 (1 H, brs), 4.116 (1 H, m), 3.888 (1 H, d, J = 10.4 Hz), 3.695 (1 H, t, J = 4.8 Hz), 3.629 (2 H, J = 1.2 Hz), 3.570–3.463 (4 H, m), 3.189 (1 H, m), 2.500–1.272 (31 H, m). 13 C-NMR (50 °C, CD 2 Cl 2 ): 170.82, 74.10, 71.52, 71.49, 70.14, 68.87, 67.95, 60.81, 57.85, 48.83, 36.88, 32.95, 32.75, 31.99, 29.91, 29.47, 29.22, 28.98, 28.62, 26.73, 26.50, 26.09, 23.06. HRMS (ESI, [M + H] + ): Calcd. For C 25 H 43 N 2 O 3 + : 419.3268, Found: 419.3296. Synthesis of 19(C11) To a solution of 14 (37.4 mg, 0.0702 mmol) in CH 2 Cl 2 (1.8 mL) was added TFA (0.3 mL), and the whole was stirred for 1 h at 0 °C and for 1.5 h at rt. The reaction mixture was poured into 10% aqueous solution of Na 2 CO 3 and the whole was extracted with CH 2 Cl 2 . The organic layer was dried over Na 2 SO 4 and evaporated. Column chromatography (AcOEt/MeOH = 20/1 to CHCl 3 /MeOH = 10/1 and 2% Et 3 N) and preparative TLC (CHCl 3 /MeOH = 16/1 and 0.2% Et 3 N) gave 19(C11) (7.2 mg, 24%) as a colorless oil. 1 H-NMR (CD 2 Cl 2 , 50 °C): 4.398 (1 H, m), 4.123(1 H, brs), 3.873 (1 H, d, J = 10.4 Hz), 3.653 (1 H, t, J = 4.8 Hz), 3.561–3.391 (6 H, m), 3.067 (1 H, m), 2.081–1.260 (33 H, m). 13 C-NMR (CD 2 Cl 2 , 50 °C): 170.97, 74.10, 71.60, 71.37, 70.06, 68.50, 67.98, 60.62, 58.23, 49.34, 36.58, 32.96, 32.48, 30.58, 30.27, 30.10, 29.88, 29.38, 29.31, 29.18, 28.72, 26.90, 26.73, 23.10. HRMS (ESI, [M + H] + ): Calcd. For C 26 H 45 N 2 O 3 + : 433.3425, Found: 433.3429. Synthesis of 20(C12) To a solution of 15 (20.4 mg, 0.03734 mmol) in CH 2 Cl 2 (0.9 mL) was added TFA (0.15 mL) and the whole was stirred for 5 h at 0 °C and evaporated. 10% Aqueous solution of Na 2 CO 3 was added to the residue to adjust the pH to 10. The whole was extracted with CH 2 Cl 2 and the combined organic layer was dried over Na 2 SO 4 and evaporated. Column chromatography (CHCl 3 /MeOH = 30/1 to 20/1 to 10/1) gave compound 20(C12) (14.9 mg, 89%) as a white solid. Mp. 98.0–99.5 °C. 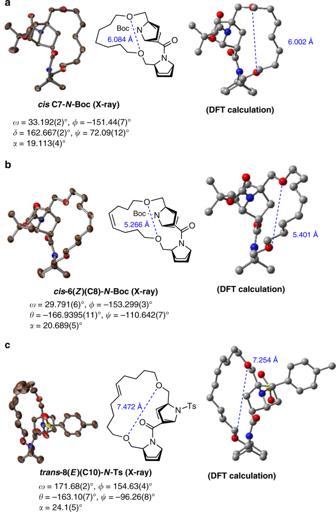Fig. 5 ORTEP drawings (50% probability) of the crystal structures of some derivatives.aThe crystal structure ofN-Boc derivative ofC7in thecisamide form.bThe crystal structure ofN-Boc derivative of6(Z) (C8) in thecis-amide form, andcthe crystal structure ofN-tosylated derivative of8(E) (Ts-8(E)(C10)) in thetrans-amide form. All three structures were crystallized as racemates in centrosymmetric space groups. DFT-optimized structures are also shown. The distance between the ether oxygen atoms in the linker is shown in blue. Brown/gray: carbon atom; blue: nitrogen atom; red: oxygen atom. All hydrogen atoms are omitted for clarity 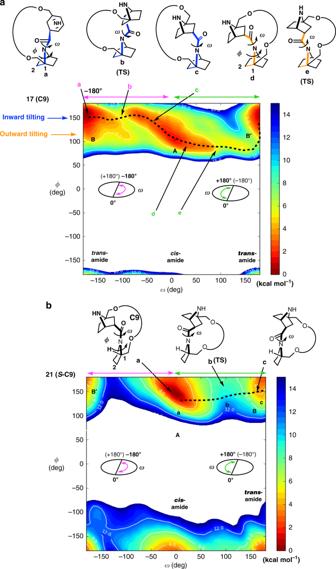Fig. 6 The landscape of lactam amide rotation.aMetadymamic simulations of bicycle lactam17(C9)in chloroform at 300 K. Dashed lines indicate the rotational pathways. The tilting direction of the pyramidal nitrogen atom of the bicyclic systems is synchronized with the direction of the semicircle-rotation of the amide.bMetadymamic simulations of monocycle lactam21(S-C9)in chloroform at 300 K. Dashed lines indicate the rotational pathways. Rotation of the lactam amide bond is restricted to a south semicircle-rotation angle (e.g., 0° to + 180°) 1 H-NMR (CD 2 Cl 2 ): 4.348 (1 H, brs), 4.053 (2 H, s), 3.663–3.644 (1 H, m), 3.575 (2 H, d, J = 9.6 Hz), 3.526–3.437 (4 H, m), 3.071–3.021 (1 H, m), 2.20–1.05 (35 H, m). 13 C-NMR (CD 2 Cl 2 ):170.82, 73.52, 71.12, 70.87, 70.06, 68.52, 68.18, 60.60, 58.42, 49.24, 35.95, 32.42, 32.33, 30.46, 30.31, 29.91, 29.72, 29.50, 29.20, 29.08, 28.31, 27.49, 26.73, 26.06. HRMS (ESI, [M + H] + ): Calcd. For C 27 H 47 N 2 O 3 + : 447.3581, Found: 447.3608. Single crystal X-ray diffraction experiment The diffraction experiments for Boc- (C7) and 6 ( Z ) (C8) were performed in a Bruker APEX II CCD detector (MoKα: λ = 0.71073 Å). Structure solution and refinement were performed by using SHELXS-97 and SHELXL-97 [42] . The diffraction experiment for Ts-8 ( E ) (C10) was performed in a Rigaku AFC7R (CuKα: λ = 1.54178 Å). Absorption correction was performed by psi-scan. Structure solution and refinement were performed with SHELXS-2013 [42] and SHELXL-2013 [43] . Metadynamics simulations Metadynamics calculations were performed with Desmond using OPSL3 force field (Schrodinger Inc., U.S.A.). The simulation conditions are as follows: Temperature = 300.0 K, Pressure = 1.01325 bar, Ensemble = NPT, Solvent = CHCl 3 .